Selective fluorescent probes for live-cell monitoring of sulphide Aqueous sulphides, including hydrogen sulphide, have important roles in biological signalling and metabolic processes. Here we develop a selective sulphide-trapping strategy involving sulphide addition to an aldehyde; the resulting hemithioacetal undergoes a Michael addition with an adjacent unsaturated acrylate ester to form a thioacetal at neutral pH in aqueous solution. Employing this new strategy, two sulphide-selective fluorescent probes, SFP-1 and SFP-2, were synthesized on the basis of two different fluorophore templates. These probes exhibit an excellent fluorescence increase and an emission maximum shift (SFP-1) in response to Na 2 S and H 2 S in a high thiol background as found under physiological conditions. We show the utility of the probes for the selective detection of sulphides, and the capacity of our probes to monitor enzymatic H 2 S biogenesis and image free sulphide in living cells. Hydrogen sulphide (H 2 S), along with nitric oxide (NO) and carbon monoxide (CO), belongs to the gasotransmitter family of signalling molecules in biology [1] , [2] . H 2 S, or aqueous sulphide, elicits diverse physiological responses, including modulation of blood pressure and reduction of ischemia reperfusion injury [3] , [4] , [5] , exertion of anti-inflammatory effects [6] and reduction of metabolic rate [7] . The production of H 2 S is catalysed by the two pyridoxal 5′-phosphate-dependent enzymes, cystathionine β-synthase (CBS) [8] , and cystathionine γ-lyase [9] , and indirectly, via a pyridoxal 5′-phosphate-independent enzyme, 3-mercaptopyruvate sulphurtransferase [10] . The lack of methods for accurate measurement of H 2 S has limited advances in the field. As a result of the technical limitations of available methods [11] , [12] , H 2 S concentrations spanning 10 5 orders of magnitude have been reported in the literature [13] . Moreover, many of the commonly used methods are not amenable for application in vivo or for analysis of tissue or blood samples. Until recently, no probe was available for the detection of aqueous sulphides in vivo (while this manuscript was under review, a related probe was reported [14] ). A major challenge is to develop molecular probes that are capable of detecting aqueous sulphides (H 2 S and HS − at neural pH) in the presence of other cellular molecules, in particular, millimolar concentrations of thiols found inside most cells. Recently, a thiol-maleimide reaction was employed to tune photoinduced electron transfer of a conjugated fluorophore for thiol detection and imaging [15] . Although effective for detection of abundant thiol molecules, this method is unable to differentiate sulphide from thiols. Partially inspired by this previous work, we envisioned an aromatic framework substituted by α, β-unsaturated acrylate methyl ester and aldehyde (–CHO) ortho to each other. The aldehyde group can react readily and reversibly with free sulphide to form a hemithioacetal intermediate with an exposed thiol, which is set up for a Michael addition to the proximal acrylate to yield a trapped thioacetal. This tandem reaction could tune photoinduced electron transfer of the aromatic system, thus potentially affecting fluorescence of a conjugated fluorophore. As reversible addition of a thiol to the same aldehyde yields a thioacetal that cannot perform the subsequent Michael addition step, the intermediate simply decomposes to yield the original probe, thus it will not significantly interfere sulphide detection. In addition, H 2 S in aqueous solution has a pK a of ~7.0, whereas thiols have higher pK a values around 8.5. Hence, aqueous sulphide is expected to be a better nucleophile at neutral pH than free thiols. In this study, we report the development of two highly sulphide-selective fluorescent probes (SFP-1 and SFP-2), using a chemical strategy for effective in vivo and in vitro detection of H 2 S. We demonstrate the utility of the probe in enzymatic H 2 S quantification and cell-based imaging applications. Synthesis and fluorescent measurements of SFP-1 We selected 1,3,5-triaryl-2-pyrazoline as the first fluorophore template because its fluorescence is sensitive to the electronic changes of the substituted aromatic groups [16] . During synthesis of the probe, we inadvertently obtained 1,3,5-triaryl-pyrazole because of a required oxidation step ( Fig. 1 ). The final probe 12 (SFP-1) was characterized by nuclear magnetic resonance (NMR), mass spectrometry and X-ray crystallography (CCDC 843032; Supplementary Figs S1–S3 , Supplementary Tables S1–S5 , Supplementary Data 1 ). The phenyl substitution at C5 of the pyrazole core is designed to react with sulphide to afford 12a ( Fig. 2 ), thus yielding a fluorescence change. 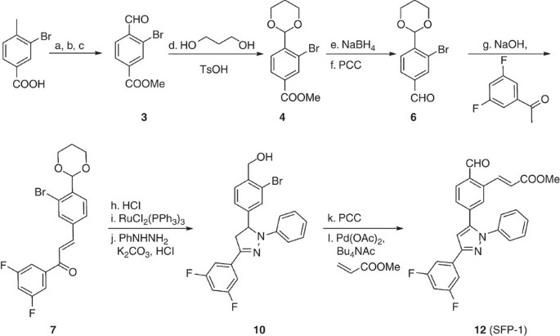Figure 1: Probe SFP-1 synthesis. (a) MeOH, H2SO4(2.0 equivalent), 80 °C, 12 h, 87%; (b) CrO3(3 equiv.), AcOH (30 equiv.), Ac2O (18 equiv.) H2SO4(4.5 equiv.) 0 °C, 1 h, 57%; (c) H2SO4, MeOH/H2O (1:1), 100 °C, 30 min, then THF, HCl, 80 °C, 2 h, 78%; (d) 1,3-propanediol (6 equiv.),p-TsOH (0.35 equiv.), anhydrous Na2SO4, 80 °C, 24 h, 80%; (e) NaBH4(10 equiv.), 1, 4-dioxane/H2O (3:2), 65 °C, 12 h, 70%; (f) PCC (1.5 equiv.), celite, CH2Cl2, 25 °C, 1 h, 90%; (g) 3′,5′-difluoroacetophenone (1.1 equiv.), 5 N NaOH (20 equiv.), EtOH, 25 °C, 2 h, 91%; (h) HCl, THF, 25 °C, 5 h, 99%; (i) RuCl2(PPh3)3(0.7% equiv.), HCOOH (2.8 equiv.), Et3N (1.7 equiv.), THF, 25 °C, 2 h, 83%; (j) phenylhydrazine (1.3 equiv.), HCl (1.3 equiv.), K2CO3(0,25 equiv.), EtOH, 90 °C, 12 h, 65%; (k) PCC (5 equiv.), celite, CH2Cl2, 25 °C, 2 h, 86%; (l) Pd(OAc)2(0.1 equiv.), methyl acrylate (1.2 equiv.), Bu4NAc (3 equiv.), K2CO3(1.5 equiv.), KCl (1.5 equiv.), DMF, 90 °C, 2 h, 56%. DMF, N,N-dimethylformamide; Et3N, triethylamine; NaBH4,sodium borohydrid; PCC, pyridinium chlorochromate; THF, tetrahydrofuran;p-TsOH,p-toluenesulfonic acid. Figure 1: Probe SFP-1 synthesis. ( a ) MeOH, H 2 SO 4 (2.0 equivalent), 80 °C, 12 h, 87%; ( b ) CrO 3 (3 equiv. ), AcOH (30 equiv. ), Ac 2 O (18 equiv.) H 2 SO 4 (4.5 equiv.) 0 °C, 1 h, 57%; ( c ) H 2 SO 4 , MeOH/H 2 O (1:1), 100 °C, 30 min, then THF, HCl, 80 °C, 2 h, 78%; ( d ) 1,3-propanediol (6 equiv. ), p -TsOH (0.35 equiv. ), anhydrous Na 2 SO 4 , 80 °C, 24 h, 80%; ( e ) NaBH 4 (10 equiv. ), 1, 4-dioxane/H 2 O (3:2), 65 °C, 12 h, 70%; ( f ) PCC (1.5 equiv. ), celite, CH 2 Cl 2 , 25 °C, 1 h, 90%; ( g ) 3′,5′-difluoroacetophenone (1.1 equiv. ), 5 N NaOH (20 equiv. ), EtOH, 25 °C, 2 h, 91%; ( h ) HCl, THF, 25 °C, 5 h, 99%; ( i ) RuCl 2 (PPh 3 ) 3 (0.7% equiv. ), HCOOH (2.8 equiv. ), Et 3 N (1.7 equiv. ), THF, 25 °C, 2 h, 83%; ( j ) phenylhydrazine (1.3 equiv. ), HCl (1.3 equiv. ), K 2 CO 3 (0,25 equiv. ), EtOH, 90 °C, 12 h, 65%; ( k ) PCC (5 equiv. ), celite, CH 2 Cl 2 , 25 °C, 2 h, 86%; ( l ) Pd(OAc) 2 (0.1 equiv. ), methyl acrylate (1.2 equiv. ), Bu 4 NAc (3 equiv. ), K 2 CO 3 (1.5 equiv. ), KCl (1.5 equiv. ), DMF, 90 °C, 2 h, 56%. DMF, N,N-dimethylformamide; Et 3 N, triethylamine; NaBH 4, sodium borohydrid; PCC, pyridinium chlorochromate; THF, tetrahydrofuran; p -TsOH, p -toluenesulfonic acid. 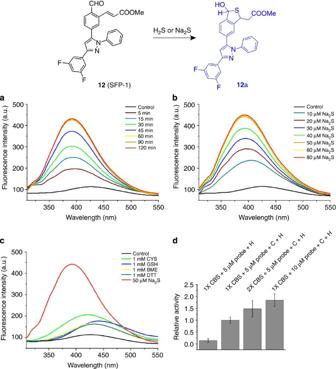Figure 2: SFP-1 reacts with sulphide to give a turn-on fluorescence response. (a–c) Fluorescence spectra of the SFP-1 probe (10 μM) in PBS buffer (10 mM, pH 7.4, 10% CH3CN) at 37 °C for 60 min. Excitation: 300 nm, emission: 310–550 nm. The data represent the average of three independent experiments. (a) Incubated with 50 μM Na2S after 5, 15, 30, 45, 60, 90 and 120 min. (b) Incubated with different concentrations of Na2S (10, 20, 30, 40, 50, 60 and 80 μM). (c) Incubated with various thiols at 1 mM (CYS, cysteine; BME, 2-mercaptoethanol; DTT, dithiothreitol). (d) Fluorescent detection of H2S generation by CBS. Human CBS was mixed with either homocysteine (H) or cysteine (C)+homocysteine (10 mM each). The H2S–producing activity of CBS in the presence of cysteine and homocysteine and 5 μM probe was set at 1 and the data represent the mean±s.d. of at least three independent experiments. Full size image Figure 2: SFP-1 reacts with sulphide to give a turn-on fluorescence response. ( a – c ) Fluorescence spectra of the SFP-1 probe (10 μM) in PBS buffer (10 mM, pH 7.4, 10% CH 3 CN) at 37 °C for 60 min. Excitation: 300 nm, emission: 310–550 nm. The data represent the average of three independent experiments. ( a ) Incubated with 50 μM Na 2 S after 5, 15, 30, 45, 60, 90 and 120 min. ( b ) Incubated with different concentrations of Na 2 S (10, 20, 30, 40, 50, 60 and 80 μM). ( c ) Incubated with various thiols at 1 mM (CYS, cysteine; BME, 2-mercaptoethanol; DTT, dithiothreitol). ( d ) Fluorescent detection of H 2 S generation by CBS. Human CBS was mixed with either homocysteine (H) or cysteine (C)+homocysteine (10 mM each). The H 2 S–producing activity of CBS in the presence of cysteine and homocysteine and 5 μM probe was set at 1 and the data represent the mean±s.d. of at least three independent experiments. Full size image Reaction of probe 12 (10 μM) with Na 2 S (50 μM) as an aqueous sulphide source at 37 °C in PBS buffer (pH 7.4) yielded a time-dependent fluorescence increase, which was completed within 60 min ( Fig. 2a, Supplementary Fig. S4 ). A >10-fold increase in the fluorescence intensity accompanied by a blue shift in the emission maximum from 428 to 391 nm was observed ( ɛ =2,320 M −1 cm −1 , Φ=0.058). Addition of sulphide most likely eliminates the quenching effects of the conjugated, unsaturated acrylate ester and aldehyde on the 5-substituted phenyl group. Consistently, a blue shift of emission indicates a break of conjugation of SFP-1 on sulphide addition. We isolated product 12a and confirmed its molecular formula by high-resolution mass spectrometry ( Supplementary Fig. S3 ). Next, varying concentrations of Na 2 S (10–50 μM) were added to the test reaction solution. The fluorescence intensity increased linearly with the concentration of Na 2 S up to 50 μM ( Supplementary Fig. S5 ), and, thereafter, reached a steady state ( Fig. 2b ). To characterize the direct response of the probe towards H 2 S, the probe was added to a buffered solution that had been bubbled with H 2 S gas. The presence of low concentrations of H 2 S led to a significant fluorescence change, confirming the utility of SFP-1 for monitoring aqueous H 2 S ( Supplementary Fig. S6 ). The specificity of the probe was examined by measuring its response after exposure to various thiols in PBS buffer. Strikingly, even at high concentrations (1 mM), the response of SFP-1 to any of the tested thiols was very low, exhibiting at least 50- to 100-fold selectivity towards sulphide ( Fig. 2c ). In addition, the emission maximum of 12a is different from those of potential thiol addition products; monitoring emission at lower wavelength should allow further distinction between sulphide versus thiol adducts. For instance, if emission can be monitored at 350 nm, the most abundant thiol in mammalian cells, glutathione, does not interfere with sulphide, thus providing potential superb selectivity for sulphide detection and imaging. To investigate whether the probe can be used to monitor enzymatic H 2 S generation, we tested its efficacy with recombinant human CBS ( Fig. 2d ). H 2 S production by CBS was readily detected in the presence of millimolar concentrations of the thiol substrates, homocysteine and/or cysteine. Doubling CBS concentration or the probe concentration (from 5 to 10 μM) resulted in increased signal intensity. These results demonstrate the excellent selectivity of the probe to H 2 S in a high thiol background and its utility as a molecular probe for detecting H 2 S biogenesis in in vitro assays. This fluorescence-based assay could be readily implemented into a high throughput format for screening compound libraries for inhibitors or activators of H 2 S production. Synthesis and fluorescent measurements of SFP-2 To further test the general applicability of the sulphide-trapping chemical strategy and to develop a fluorescent probe with visible-wavelength excitation and emission, we employed 4,4-Difluoro-1,3,5,7-tetramethyl-4-bora-3a,4a-diaza-s-indacene (BODIPY) as the second fluorophore template owing to its high brightness and photostability [17] . 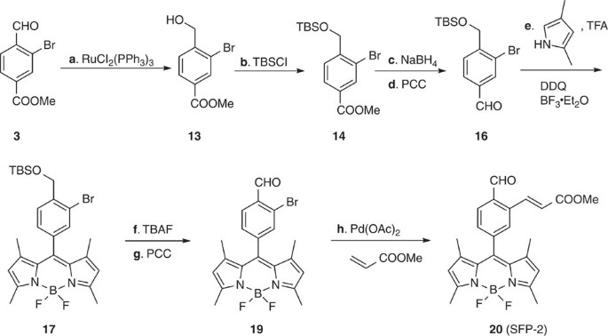Figure 3: Probe SFP-2 synthesis. (a) RuCl2(PPh3)3(0.7% equivalent), HCOOH (2.8 equiv.), Et3N (1.7 equiv.), THF, 25 °C, 2 h, 92%; (b) TBSCl (1.2 equiv.), imidazole (2 equiv.), DMF, 25 °C, 12 h, 99%; (c) NaBH4(10 equiv.), 1, 4-dioxane/H2O (3:2), 65 °C, 12 h, 72%; (d) PCC (1.5 equiv.), celite, CH2Cl2, 25 °C, 1 h, 64%; (e) (1) 2,4-dimethylpyrrole (2 equiv.), TFA (one drop), CH2Cl2, 25 °C, 12 h. (2) DDQ (1 equiv.), CH2Cl2, 25 °C, 1 h. (3) DIPEA (10 equiv.), BF3·Et2O (30 equiv.), CH2Cl2, 25 °C, 2 h, 58%; (f) TBAF (1 equiv.), THF, 25 °C, 30 min, 83%; (g) PCC (5 equiv.), MgSO4, CH2Cl2, 25 °C, 30 min, 65%; (h) Pd(OAc)2(0.1 equiv.), methyl acrylate (4 equiv.), PPh3(0.3 equiv.), Et3N (1.5 equiv.), CH3CN, 90 °C, 12 h, 38%. DDQ, 2,3-Dichloro-5,6-dicyano-p-benzoquinone; DIPEA , N, N-Diisopropylethylamine; DMF, N,N-dimethylformamide; Et3N, triethylamine; NaBH4,sodium borohydrid; PCC, pyridinium chlorochromate; TBAF, Tetrabutylammonium fluoride trihydrate; TBSCl, tert-Butyl(chloro)dimethylsilane; TFA, Trifluoroacetic acid; THF, tetrahydrofuran. We synthesized the BODIPY-based probe SFP-2 ( 20 ) as shown in Figure 3 . The final probe 20 (SFP-2) was characterized by NMR and mass spectrometry ( Supplementary Fig. S7 ). We expected a turn-on response of the probe after reacting with sulphide to afford 20a ( Fig. 4 ). We also isolated product 20a and confirmed its molecular formula by high-resolution mass spectrometry ( Supplementary Fig. S8 ). We evaluated this new SFP-2 probe (5 μM) with Na 2 S (50 μM) as an aqueous sulphide source at 37 °C in 20 mM PBS buffer (pH 7.0) ( Fig. 4a , Supplementary Fig. S9 ). SFP-2 showed a >13-fold increase of the fluorescence intensity in the emission maximum at 510 nm when excited at 465 nm ( ɛ =47,100 M −1 cm −1 , Φ=0.208). The high optical brightness of the probe allows for detection of free sulphide without undergoing the full intensity change. Figure 3: Probe SFP-2 synthesis. ( a ) RuCl 2 (PPh 3 ) 3 (0.7% equivalent), HCOOH (2.8 equiv. ), Et 3 N (1.7 equiv. ), THF, 25 °C, 2 h, 92%; ( b ) TBSCl (1.2 equiv. ), imidazole (2 equiv. ), DMF, 25 °C, 12 h, 99%; ( c ) NaBH 4 (10 equiv. ), 1, 4-dioxane/H 2 O (3:2), 65 °C, 12 h, 72%; ( d ) PCC (1.5 equiv. ), celite, CH 2 Cl 2 , 25 °C, 1 h, 64%; ( e ) (1) 2,4-dimethylpyrrole (2 equiv. ), TFA (one drop), CH 2 Cl 2 , 25 °C, 12 h. (2) DDQ (1 equiv. ), CH 2 Cl 2 , 25 °C, 1 h. (3) DIPEA (10 equiv. ), BF 3 ·Et 2 O (30 equiv. ), CH 2 Cl 2 , 25 °C, 2 h, 58%; ( f ) TBAF (1 equiv. ), THF, 25 °C, 30 min, 83%; ( g ) PCC (5 equiv. ), MgSO 4 , CH 2 Cl 2 , 25 °C, 30 min, 65%; ( h ) Pd(OAc) 2 (0.1 equiv. ), methyl acrylate (4 equiv. ), PPh 3 (0.3 equiv. ), Et 3 N (1.5 equiv. ), CH 3 CN, 90 °C, 12 h, 38%. DDQ, 2,3-Dichloro-5,6-dicyano- p -benzoquinone; DIPEA , N, N-Diisopropylethylamine; DMF, N,N-dimethylformamide; Et 3 N, triethylamine; NaBH 4, sodium borohydrid; PCC, pyridinium chlorochromate; TBAF, Tetrabutylammonium fluoride trihydrate; TBSCl, tert-Butyl(chloro)dimethylsilane; TFA, Trifluoroacetic acid; THF, tetrahydrofuran. 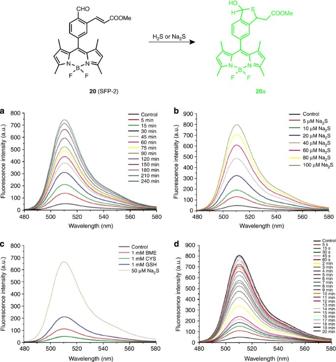Figure 4: SFP-2 reacts with sulphide to give a turn-on fluorescence response. (a–c) Fluorescence spectra of the SFP-2 probe (5 μM) in PBS buffer (20 mM, pH 7.0, 1% DMSO) at 37 °C. Excitation: 465 nm, emission: 480–580 nm. The data represent the average of three independent experiments. (a) Incubated with 50 μM Na2S after 5, 15, 30, 45, 60, 75, 90, 120, 150, 180 and 240 min. (b) Incubated with different concentrations of Na2S (5, 10, 20, 40, 60, 80 and 100 μM) for 120 min. (c) Incubated with various thiols at 1 mM (BME, 2-mercaptoethanol; CYS, cysteine; GSH, glutathione) for 180 min. (d) Incubated with 1 μl H2S buffer (bubbling H2S 10 min–saturated solution) at 25 °C from 5 s–20 min. Full size image Figure 4: SFP-2 reacts with sulphide to give a turn-on fluorescence response. ( a – c ) Fluorescence spectra of the SFP-2 probe (5 μM) in PBS buffer (20 mM, pH 7.0, 1% DMSO) at 37 °C. Excitation: 465 nm, emission: 480–580 nm. The data represent the average of three independent experiments. ( a ) Incubated with 50 μM Na 2 S after 5, 15, 30, 45, 60, 75, 90, 120, 150, 180 and 240 min. ( b ) Incubated with different concentrations of Na 2 S (5, 10, 20, 40, 60, 80 and 100 μM) for 120 min. ( c ) Incubated with various thiols at 1 mM (BME, 2-mercaptoethanol; CYS, cysteine; GSH, glutathione) for 180 min. ( d ) Incubated with 1 μl H 2 S buffer (bubbling H 2 S 10 min–saturated solution) at 25 °C from 5 s–20 min. Full size image We further examined the sensitivity of SFP-2 for sulphide. The fluorescent intensity increased by 2.6–16 folds with addition of 5–100 μM Na 2 S ( Fig. 4b ; Supplementary Figs S10, S11 ). The turn-on fluorescence response is also highly selective for sulphide versus various biological relevant thiols in the PBS buffer ( Fig. 4c ). The SFP-2 probe is ~260-fold more selective towards Na 2 S than to cysteine, and ~150-fold more selective for Na 2 S than for glutathione. Direct response towards H 2 S was also tested. After addition of 1 μl H 2 S buffered solution (10 min H 2 S bubbling), a significant fluorescence increase was observed after 5 s to 20 min of mixing, and the reaction was complete in 20 min at 25 °C ( Fig. 4d ). A smaller amount of H 2 S can still induce a significant response, further confirming that SFP-2 probe is a sensitive and selective probe for H 2 S detection ( Supplementary Fig. S12 ). Cellular imaging experiments Additionally, we tested the utility of both probes for live-cell imaging of sulphide. Even at high concentrations of SFP-1 (50 μM), adverse effects of the probe on cell viability were minimal ( Supplementary Fig. S13 ). HeLa cells were incubated with either probe for 15 min before replacing the culture medium with fresh medium containing varying concentrations of Na 2 S. Whereas some background fluorescence was observed even in the absence of added sulphide for 10 μM of SFP-1 ( Fig. 5a ), the signal intensity increased as the concentration of sulphide was increased from 10 to 100 μM ( Fig. 5b–d ). SFP-2 (2 μM) responded at slightly higher concentrations of Na 2 S, with the sulphide concentration ranging from 0 to 200 μM ( Fig. 5e–h ). However, SFP-2 is a brighter probe and excites and emits at visible range that is desirable for cell-based imaging. These results demonstrate that these probes are selective for sulphide and amenable for live-cell imaging. 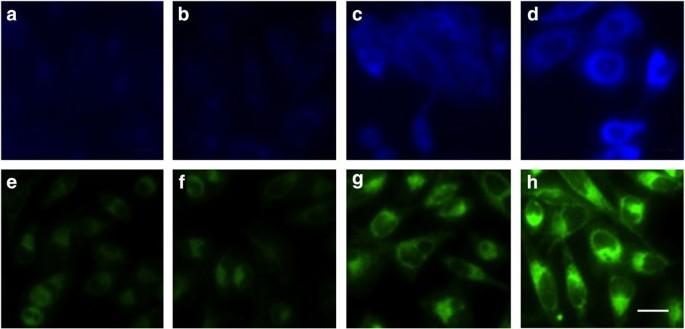Figure 5: Response of the probes with increasing concentrations of Na2S. (a–d) Imaging of aqueous sulphide in HeLa cells after 15 min incubation using SFP-1 (12) or SFP-2 (20). For12, excitation and data collection were performed using the corresponding filters for DAPI (blue) on a DSU spinning disk confocal. For20, similar experiments were performed using the filter for green fluorescent protein (green). Images were obtained by using widefield fluorescence capture with SFP-1 (10 μM), with increasing concentrations of Na2S: (a) 0 μM, (b) 10 μM, (c) 50 μM, and (d) 100 μM. With SFP-2 (2 μM), confocal fluorescence capture was utilized, and Na2S concentrations were varied from (e) 0 μM, (f) 50 μM, (g) 100 μM, and (h) 200 μM. Scale bar represents 20 μm. Figure 5: Response of the probes with increasing concentrations of Na 2 S. ( a – d ) Imaging of aqueous sulphide in HeLa cells after 15 min incubation using SFP-1 ( 12 ) or SFP-2 ( 20 ). For 12 , excitation and data collection were performed using the corresponding filters for DAPI (blue) on a DSU spinning disk confocal. For 20 , similar experiments were performed using the filter for green fluorescent protein (green). Images were obtained by using widefield fluorescence capture with SFP-1 (10 μM), with increasing concentrations of Na 2 S: ( a ) 0 μM, ( b ) 10 μM, ( c ) 50 μM, and ( d ) 100 μM. With SFP-2 (2 μM), confocal fluorescence capture was utilized, and Na 2 S concentrations were varied from ( e ) 0 μM, ( f ) 50 μM, ( g ) 100 μM, and ( h ) 200 μM. Scale bar represents 20 μm. Full size image In addition to supplementing cells with extraneous sources of sulphide, we sought to determine whether we could detect intrinsically produced H 2 S by perturbing the pool of precursors to H 2 S biosynthesis inside the cell. The amino acid cysteine and glutathione (reduced) (GSH) can both serve as potential sulphide sources. The previously mentioned enzymes, CBS and cystathionine γ-lyase, both use cysteine as a substrate for H 2 S production [8] , [9] , [18] , [19] , [20] . GSH can be broken down by γ-glutayml transpeptidase and a dipeptidase to give cysteine [21] , [22] , [23] , which can then be converted to H 2 S. Therefore, we tested whether a perturbation of the intracellular levels of either cysteine, or GSH could result in an increased cellular concentration of H 2 S. Imaging experiments were carried out with SFP-2, as previously described, and cells were incubated with either 100 μM GSH or cysteine. After 30 min of incubation, addition of both thiol species elicited a significant response rivalling that observed for Na 2 S ( Fig. 6 ). Other biologically relevant sulphur sources, including a thioether and a disulphide, did not generate a similar response ( Supplementary Fig. S14 ). These results further indicate that these probes are capable of detecting not only external sulphides supplemented to cell cultures, but also sulphides biologically produced by the cells. 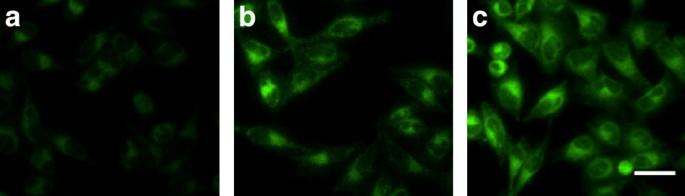Figure 6: Response of SFP-2 using different thiol substrates. (a–c) Imaging of sulphide substrates in HeLa cells after 30 min incubation using SFP-2 (20). Images were obtained by using confocal fluorescence capture with 2 μM probe, with either: (a) 0 μM sulphide source, (b) 100 μM GSH, (c) 100 μM cysteine. Scale bar represents 40 μm. Figure 6: Response of SFP-2 using different thiol substrates. ( a – c ) Imaging of sulphide substrates in HeLa cells after 30 min incubation using SFP-2 ( 20 ). Images were obtained by using confocal fluorescence capture with 2 μM probe, with either: ( a ) 0 μM sulphide source, ( b ) 100 μM GSH, ( c ) 100 μM cysteine. Scale bar represents 40 μm. Full size image To generate a significant response for both SFP-1 and SFP-2, higher concentrations of Na 2 S are required for the live-cell imaging experiments than the in vitro experiments. We reason that sodium sulphide, with its high charge density, could have difficulty passing through the cell membrane. The addition of this extraneous sulphide may lead to a much smaller fluctuation of the free sulphide level inside cells. With GSH and cysteine, 1 mM of either thiol gave a very weak response for SFP-1 and SFP-2 in vitro ( Figs 2c and 4c ), whereas only 100 μM of each elicited a significant response approximating that of Na 2 S in vivo . Considering the inability of the probe to detect cysteine or GSH in vitro and the millimolar concentrations of thiols already existing inside cells, we believe the response is a result of the free sulphide generated intracellularly owing to a response to the perturbed cellular levels of cysteine or GSH. We suspect that supplementing extra amounts of glutathione may disrupt glutathione homeostasis and H 2 S biogenesis, leading to an increased level of H 2 S. Thus, the probe shows great promise as a reporter for monitoring sulphide fluctuation inside cells, and could help elucidating pathways for sulphide production and uncovering new genes responsible for sulphide homeostasis. The development of innovative fluorescent imaging probes has revolutionized cell biology, allowing localization and dynamic monitoring of cellular metabolite and inorganic ion pools [15] , [16] , [24] , [25] , [26] , [27] , [28] , [29] . A significant bottleneck in the emerging field of H 2 S/aqueous sulphide signalling is the absence of technology for effective in vivo detection and imaging, a problem that is exacerbated by the high intracellular thiol concentration. In this study, we have successfully developed a chemical strategy for selective sulphide detection, which can be used to monitor sulphide generation from enzymes and for cell-based sulphide imaging in live cells in the presence of large excess of thiols. Tandem chemical reactions, consisted of a sulphide addition to an aldehyde and the resulting hemithioacetal performing a Michael addition to an unsaturated acrylate ester to form a thioacetal at neutral pH in aqueous solution, provide the basis for the sulphide selectivity. We show that the same chemistry can be readily adapted to different fluorescent templates for sulphide detection and imaging. The same chemistry will lead to new probes with faster response, which may help to monitor fluctuations of H 2 S in situ . Further optimization and utilization of this strategy and this class of probes should dramatically accelerate future studies of H 2 S in biology. Probe synthesis Detailed description of the synthesis of each probe can be found in the Supplementary Methods . Each step was characterized by thin-layer chromatography, high-resolution mass spectra, and both 1 H and 13 C NMR ( Supplementary Figs S15–S54 ). Fluorometric analysis All fluorescence measurements were carried out at room temperature on a Varian Cary Eclipse fluorescence spectrophotometer. Samples were excited at 300 and 465 nm with the excitation and emission slit widths set at 5 and 10 nm for SFP-1 and SFP-2, respectively. The emission spectrum was scanned from 310 to 550 nm and from 480 to 580 nm at 120 nm min −1 , respectively. The photomultiplier voltage was set at 1,000 V for SFP-1 and 600 V for SFP-2. The probe was dissolved in CH 3 CN or dimethylsulphoxide (DMSO) to make a 10 mM stock solution, which was diluted to the required concentration for measurement. Cytotoxicity assay HeLa cells were grown up in DMEM media with 10% FBS and penicillin/streptomycin (Invitrogen). Cells were allowed to grow to 80% confluency before being collected using trypsin-EDTA. The cell number was determined and solution was diluted to a final concentration of 2.22×10 5 cells ml −1 in the aforementioned media. A final number of 2×10 4 cells (90 μl) was transferred to each well in a 96-well plate (BD Falcon). Cells were incubated overnight at 37 °C in a 5% CO 2 atmosphere. A serial dilution on SFP-1 was performed in DMEM media, with 10 μl added to each well to give final concentrations of 0.4, 0.8, 1.6, 3.1, 12.5, 25, 50 and 100 μM probe. Cells were allowed to incubate for 20 h. Wells containing only cells and only probe were also set up to serve as positive and negative controls. Dye solution and stop/solubilization mix were obtained from a CellTiter 96 non-radioactive cell proliferation assay (Promega). Cytotoxicity assay was performed as per manufacturer's instructions. Absorbance at 570 was monitored using a Synergy plate reader (Biotek). Data was collected for three separate serial dilutions and averaged. Cellular imaging experiments HeLa cells were grown, as previously described. Cells were allowed to grow to 80% confluency before being collected and transferred to a 6-well plate (BD Falcon). These cells were allowed to grow overnight at 37 °C in a 5% CO 2 atmosphere. Cells were maintained at these conditions until immediately before imaging experiments. At this time, a final concentration of 10 μM SFP-1 or 2 μM SFP-2 was added to the cells and they were allowed to incubate at the previous conditions for 15 min. Media was then removed, and fresh media was added to remove any probe left in solution and optimize the background signal. The sulphur source was then added (Na 2 S, cysteine, or GSH) to the desired concentration and cells were incubated for 15–30 min at room temperature before imaging. All imaging experiments were performed on a fixed cell DSU spinning confocal microscope (Olympus). Widefield fluorescence capture was used to visualize SFP-1 under all conditions. Excitation and emission monitored using the 4′,6-diamidino-2-phenylindole dihydrochloride (DAPI) filters provided with the scope, set at 387 per 11 nm and 440 per 40 nm, respectively. Confocal fluorescence capture was used to visualize SFP-2. Excitation and emission were monitored using green filter provided with the scope, set at 485 per 20 nm and 525 per 30 nm, respectively. Imaging performed using either the X20 or X40 dry objectives that are provided with the scope. Images were captured using Slidebook software. How to cite this article: Qian, Y. et al . Selective fluorescent probes for live-cell monitoring of sulphide. Nat. Commun. 2:495 doi: 10.1038/ncomms1506 (2011).